miR-205 acts as a tumour radiosensitizer by targeting ZEB1 and Ubc13 Tumour cells associated with therapy resistance (radioresistance and drug resistance) are likely to give rise to local recurrence and distant metastatic relapse. Recent studies revealed microRNA (miRNA)-mediated regulation of metastasis and epithelial–mesenchymal transition; however, whether specific miRNAs regulate tumour radioresistance and can be exploited as radiosensitizing agents remains unclear. Here we find that miR-205 promotes radiosensitivity and is downregulated in radioresistant subpopulations of breast cancer cells, and that loss of miR-205 is highly associated with poor distant relapse-free survival in breast cancer patients. Notably, therapeutic delivery of miR-205 mimics via nanoliposomes can sensitize the tumour to radiation in a xenograft model. Mechanistically, radiation suppresses miR-205 expression through ataxia telangiectasia mutated (ATM) and zinc finger E-box binding homeobox 1 (ZEB1). Moreover, miR-205 inhibits DNA damage repair by targeting ZEB1 and the ubiquitin-conjugating enzyme Ubc13. These findings identify miR-205 as a radiosensitizing miRNA and reveal a new therapeutic strategy for radioresistant tumours. Radiotherapy is one of the major modalities of cancer treatment. A main reason of failure in radiation treatment is intrinsic and therapy-induced radioresistant tumour cells, which display enhanced DNA repair ability [1] . Combining chemotherapy with radiation improves outcomes but often increases toxicity [2] . To overcome this problem, it is necessary to elucidate the mechanisms of resistance to radiotherapy and develop new radiosensitizers. A growing number of studies have demonstrated that tumour initiation and progression can be regulated by microRNAs (miRNAs) [3] , [4] , [5] , [6] , which are small non-coding RNAs acting as negative regulators of gene expression [7] . Whereas no miRNAs have been approved by the FDA (Food and Drug Administration) as drugs, much progress is being made in developing them as therapeutic strategies [8] , [9] , [10] . For instance, locked nucleic acid-based miR-122 antagonist has shown therapeutic benefits in a phase 2 clinical trial to treat patients with hepatitis C virus infection [11] . Moreover, we and others have demonstrated the efficacy of miRNA-based therapeutic agents in preclinical models of cancer [12] , [13] , [14] . Notably, MRX34, a liposomal miR-34 mimic, entered phase 1 clinical trials in patients with advanced liver cancer in April 2013, representing the first miRNA-based drug used in cancer trials [10] . Recently, several miRNAs have been found to regulate DNA damage response in cell culture systems [15] , [16] , [17] , [18] , [19] , [20] . However, whether specific miRNAs control tumour radioresistance in vivo and can be used as tumour radiosensitizers remains unclear. In this study, we show that miR-205 is downregulated in radioresistant subpopulations of breast cancer cells derived from ionizing radiation (IR) in an ATM- and ZEB1-dependent manner. We further demonstrate the therapeutic utility of the nanoliposome-encapsulated miR-205 mimic as a tumour radiosensitizer in a preclinical model. Mechanistically, miR-205 inhibits DNA damage repair and radiosensitizes tumor cells by targeting ZEB1 and Ubc13. These results suggest that delivery of miR-205 combined with radiotherapy may represent a new strategy for cancer treatment. miR-205 negatively correlates with radioresistance To establish a radioresistant model, we used γ-IR to select the radioresistant subpopulation (designated as SUM159-P2 cells) from the parental SUM159 human breast cancer cell line ( Fig. 1a ). Irradiation is known to cause DNA double-strand breaks (DSBs), which lead to the formation of γH2AX foci, and the persistent presence of γH2AX foci indicates delayed repair and is associated with radiosensitivity [21] , [22] , [23] . At 24 h after irradiation, γH2AX foci remained in the parental SUM159 (SUM159-P0) cells but disappeared in SUM159-P2 cells ( Supplementary Fig. 1a ), suggesting that this radioresistant subline has enhanced ability to clear DNA breaks. 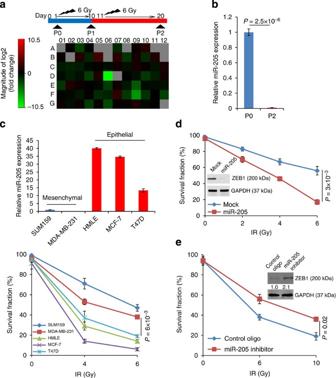Figure 1: miR-205 increases radiosensitivity and is downregulated in radioresistant breast cancer cells. (a) Top: schematic representation of the generation of a radioresistant subline (SUM159-P2) from the parental SUM159 cells (SUM159-P0). Bottom: miRNA expression profiling of SUM159-P2 cells relative to SUM159-P0 cells using a quantitative PCR (qPCR)-based miRNA array. The expression values are shown inSupplementary Table 1. (b) TaqMan qPCR analysis of miR-205 in SUM159-P0 and SUM159-P2 cells.n=3 samples per group. (c) qPCR of miR-205 (top) and clonogenic survival assays (bottom) of mesenchymal-like and epithelial-like breast cancer cell lines.n=3 samples per group. (d) Clonogenic survival assays of SUM159-P2 cells transduced with miR-205.n=3 wells per group. (e) Clonogenic survival assays of SUM159-P0 cells transfected with the miR-205 inhibitor.n=3 wells per group. Inset ind,e: immunoblotting of ZEB1 and GAPDH. Data inb–eare the mean of biological replicates from a representative experiment, and error bars indicate s.e.m. Statistical significance was determined by a two-tailed, unpaired Student’st-test. The experiments were repeated three times. Figure 1: miR-205 increases radiosensitivity and is downregulated in radioresistant breast cancer cells. ( a ) Top: schematic representation of the generation of a radioresistant subline (SUM159-P2) from the parental SUM159 cells (SUM159-P0). Bottom: miRNA expression profiling of SUM159-P2 cells relative to SUM159-P0 cells using a quantitative PCR (qPCR)-based miRNA array. The expression values are shown in Supplementary Table 1 . ( b ) TaqMan qPCR analysis of miR-205 in SUM159-P0 and SUM159-P2 cells. n =3 samples per group. ( c ) qPCR of miR-205 (top) and clonogenic survival assays (bottom) of mesenchymal-like and epithelial-like breast cancer cell lines. n =3 samples per group. ( d ) Clonogenic survival assays of SUM159-P2 cells transduced with miR-205. n =3 wells per group. ( e ) Clonogenic survival assays of SUM159-P0 cells transfected with the miR-205 inhibitor. n =3 wells per group. Inset in d , e : immunoblotting of ZEB1 and GAPDH. Data in b – e are the mean of biological replicates from a representative experiment, and error bars indicate s.e.m. Statistical significance was determined by a two-tailed, unpaired Student’s t -test. The experiments were repeated three times. Full size image We wanted to use an unbiased approach to identify miRNAs that regulate radiosensitivity. To this end, we performed a human apoptosis miRNA PCR array analysis to identify miRNAs deregulated in SUM159-P2 cells. Although most of the miRNAs on this array showed no substantial difference (fold change <2), miR-205 stood out as a miRNA that was dramatically downregulated in SUM159-P2 cells compared with the parental SUM159 cells (fold change=1,439, Fig. 1a and Supplementary Table 1 ). Individual TaqMan quantitative PCR assays further confirmed this array result ( Fig. 1b ). Recently, cancer stem cells, which are defined operationally as tumour-initiating cells, have been found to promote radioresistance through activation of DNA damage response [24] , [25] , [26] , [27] . Moreover, a transdifferentiation process, termed epithelial–mesenchymal transition (EMT), has been shown to generate cells with properties of stem cells or cancer stem cells [28] . Interestingly, miR-205 can suppress EMT by targeting the EMT-inducing transcription factor ZEB1 (ref. 29 ). We therefore reasoned that this miRNA may be negatively associated with radioresistance. Indeed, when compared with epithelial-like breast cancer cell lines, mesenchymal-like breast cancer cell lines exhibited much lower levels of miR-205 and higher clonogenic survival ability after irradiation ( Fig. 1c ). Next we performed gain-of-function and loss-of-function analyses of miR-205. The overexpression of miR-205 in SUM159-P2 cells downregulated ZEB1 and sensitized these cells to radiation ( Fig. 1d ). Conversely, the transfection of SUM159-P0 cells with the miR-205 antisense inhibitor upregulated ZEB1 and conferred radioresistance on these cells ( Fig. 1e ). Similar effects were also observed in MDA-MB-231 breast cancer cells ( Supplementary Fig. 1b ). In addition, overexpression of miR-205 rendered the A549 human lung cancer cells and the U2OS human osteosarcoma cells more radiosensitive ( Supplementary Fig. 1c,d ). Thus, the observed effect of miR-205 is not limited to the SUM159 breast cancer cell line. Therapeutic delivery of miR-205 radiosensitizes tumours Cancer cells associated with therapy resistance (radioresistance and drug resistance) are likely to be a source for tumor recurrence and distant relapse (metastasis) [30] . To investigate the clinical relevance of miR-205 expression levels, we performed a retrospective analysis on a cohort of human breast cancer patients (Oxford collection) in which miRNA profiling was obtained from 207 tumor samples; 84% of these patients received radiotherapy [31] , [32] . This analysis revealed that patients with low miR-205 expression levels (defined as the bottom 20%) in their tumours had much worse distant relapse-free survival than those with high miR-205 expression levels (defined as the top 20%; P =0.006, Fig. 2a ). 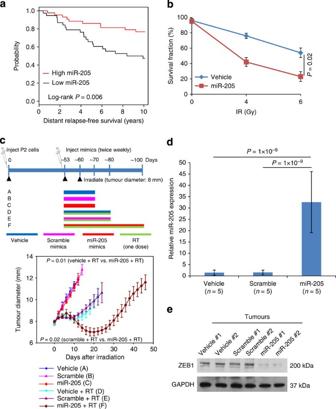Figure 2: Therapeutic effect of miR-205 mimics in mice. (a) Kaplan–Meier curves showing the distant relapse-free survival of patients with high (n=43) or low (n=38) expression of miR-205 in their breast tumours. ThePvalue was determined by a log-rank test. (b) Clonogenic survival assays of SUM159-P2 cells incubated with 100 nM DOPC-encapsulated miR-205 mimics.n=3 wells per group. (c) Top: overview of the experimental scheme. Bottom: tumour size of mice bearing SUM159-P2 xenografts. Mice were treated with the vehicle or DOPC-encapsulated miR-205 mimics or scramble mimics. Tumours were locally irradiated with a 15-Gy single dose (radiation treatment).n=5 mice per group. General linear model multivariate analysis was performed to determine statistical significance. (d) Quantitative PCR of miR-205 in tumour tissues from the mice described inc.n=5 mice per group. (e) Immunoblotting of ZEB1 and GAPDH in tumour lysates. Data inb–dare the mean of biological replicates from a representative experiment, and error bars indicate s.e.m. Statistical significance inb,dwas determined by a two-tailed, unpaired Student’st-test. The experiments were repeated three times. Figure 2: Therapeutic effect of miR-205 mimics in mice. ( a ) Kaplan–Meier curves showing the distant relapse-free survival of patients with high ( n =43) or low ( n =38) expression of miR-205 in their breast tumours. The P value was determined by a log-rank test. ( b ) Clonogenic survival assays of SUM159-P2 cells incubated with 100 nM DOPC-encapsulated miR-205 mimics. n =3 wells per group. ( c ) Top: overview of the experimental scheme. Bottom: tumour size of mice bearing SUM159-P2 xenografts. Mice were treated with the vehicle or DOPC-encapsulated miR-205 mimics or scramble mimics. Tumours were locally irradiated with a 15-Gy single dose (radiation treatment). n =5 mice per group. General linear model multivariate analysis was performed to determine statistical significance. ( d ) Quantitative PCR of miR-205 in tumour tissues from the mice described in c . n =5 mice per group. ( e ) Immunoblotting of ZEB1 and GAPDH in tumour lysates. Data in b – d are the mean of biological replicates from a representative experiment, and error bars indicate s.e.m. Statistical significance in b , d was determined by a two-tailed, unpaired Student’s t -test. The experiments were repeated three times. Full size image To determine the therapeutic potential of miR-205 as a tumour radiosensitizer, we incorporated miR-205 mimics or the scramble mimics into nanoparticles, the neutral liposome 1,2-dioleoyl-sn-glycero-3-phosphatidylcholine (DOPC), which has been shown to remain in various organs of injected animals for at least 48 h with no detectable toxicity [33] . Notably, DOPC-mediated delivery of specific short interfering RNA (siRNA) or miRNA oligonucleotides injected twice weekly at a dose of 150–200 μg kg −1 body weight yielded efficient in vivo delivery and significant antitumour effects [34] , [35] , [36] . We incubated SUM159-P2 cells with 100 nM DOPC-encapsulated miR-205 mimics for 48 h and assessed the effect on radioresistance in vitro . When compared with the vehicle control, cells treated with miR-205 mimics displayed a 57% reduction in clonogenic survival ( Fig. 2b and Supplementary Fig. 2a,b ). Subsequently, we performed therapeutic studies in mice bearing SUM159-P2 xenograft tumours. We administered miR-205 mimics subcutaneously near the tumour, because: (i) in a phase 2 clinical trial to treat patients with hepatitis C virus infection, subcutaneous injection of the anti-miR-122 locked nucleic acid (miravirsen, Santaris Pharma A/S) provided robust dose-dependent antiviral acitivity [11] ; and (ii) in mice implanted with PC-3 prostate cancer cells, subcutaneous injection of liposomal siRNA targeting BCL2 around the tumour strongly inhibited tumour growth [37] . When the SUM159-P2 tumor reached 8 mm in diameter, we locally irradiated the tumour with a 15-Gy single dose; 1 week before radiation treatment, we started the twice-weekly treatment with PBS, the scramble mimics or miR-205 mimics (250 μg kg −1 ) until the tumour burden or body condition reached the euthanasia criteria ( Fig. 2c ). Whereas radiation treatment alone led to a short initial response, treatment with miR-205 mimics alone (without tumour irradiation) had no effect on tumor size ( Fig. 2c ). In contrast, in mice with irradiated tumours, subcutaneous injection of nanoliposomal miR-205 mimics close to the tumour, which increased miR-205 levels in the tumour by approximately 21-fold ( Fig. 2d ), significantly delayed tumour growth compared with the vehicle control ( P =0.01) or scramble mimics ( P =0.02; Fig. 2c ). Consistent with increased miR-205 levels, ZEB1 protein in the tumour was markedly downregulated by treatment with miR-205 mimics ( Fig. 2e ). Histopathological examination revealed massively increased necrosis in tumours treated with both miR-205 mimics and radiation ( Supplementary Fig. 2c ), whereas the liver displayed no necrosis, steatosis or fibrosis in any group; similarly, no pathological changes were found in the kidney ( Supplementary Fig. 2d ). Taken together, these results indicate that the nanoparticle-mediated delivery of miR-205 mimics can sensitize tumours to localized irradiation but does not affect non-irradiated tumours or other organs. miR-205 inhibits radioresistance by targeting ZEB1 and Ubc13 We attempted to understand how miR-205 enhances radiosensitivity. After IR treatment, γH2AX foci persist longer in radiosensitive cells than in radioresistant cells [23] . In miR-205-overexpressing SUM159-P2 cells but not in cells infected with a scramble control, we observed persistent presence of γH2AX foci 24 h after exposure to 6-Gy IR ( Fig. 3a ), indicating that these miR-205-overexpressing cells were less able to repair DNA lesions. A critical pathway involved in DSB repair is the homologous recombination (HR) pathway [38] . We used a U2OS stable clone with chromosomal integration of an HR repair reporter containing two differentially mutated green fluorescent protein (GFP) genes (SceGFP and iGFP) oriented as direct repeats (DR-GFP); I-SceI endonuclease can generate a site-specific DSB in the SceGFP coding region, and if this DSB is repaired by HR, the expression of GFP is restored and can be quantitated by flow cytometry [39] , [40] . We observed that on I-SceI expression, miR-205-overexpressing U2OS cells exhibited an approximately 80% decrease in the percentage of GFP-positive cells, which indicated defective HR repair ( Fig. 3b ). Recently, we found that ZEB1 promotes radioresistance and HR repair through CHK1 (ref. 41 ). In the present study, re-expression of ZEB1 in miR-205-overexpressing U2OS cells partially (~30%) restored HR-based repair ( Fig. 3b and Supplementary Fig. 3a ), suggesting that ZEB1 mediates in part the effect of miR-205 on HR repair, but other functional targets of miR-205 may also be involved. 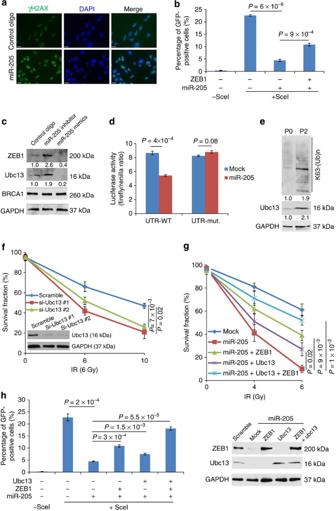Figure 3: miR-205 regulates DNA damage repair and radiosensitivity through ZEB1 and Ubc13. (a) γH2AX and 4',6-diamidino-2-phenylindole (DAPI) staining of SUM159-P2 cells transfected with miR-205 or scramble control oligonucleotides, 24 h after 6-Gy IR. Scale bar, 20 μm. (b) HR repair assays of U2OS_DR-GFP cells transfected with miR-205 alone or in combination with ZEB1.n=3 wells per group. (c) Immunoblotting of ZEB1, Ubc13, BRCA1 and GAPDH in SUM159-P0 cells transfected with miR-205 mimics or the miR-205 inhibitor. (d) Luciferase activity of the wild-type (UTR-WT) or mutant (UTR-mut.)Ubc133′ UTR reporter gene in 293T cells transfected with the miR-205-expressing or empty vector.n=3 wells per group. (e) Immunoblotting of K63-linked polyubiquitin chains, Ubc13 and GAPDH in SUM159-P0 and SUM159-P2 cells. (f) Clonogenic survival assays of SUM159-P2 cells transfected with Ubc13 siRNA.n=3 wells per group. (g) Top: clonogenic survival assays of miR-205-transduced SUM159-P2 cells with or without ectopic expression of ZEB1 and Ubc13. Bottom: immunoblotting of ZEB1, Ubc13 and GAPDH.n=3 wells per group. (h) HR repair assays of U2OS_DR-GFP cells transfected with miR-205 alone or in combination with ZEB1 or Ubc13, or both.n=3 wells per group. Data inb,d,f,g,hare the mean of biological replicates from a representative experiment, and error bars indicate s.e.m. Statistical significance was determined by a two-tailed, unpaired Student’st-test. The experiments were repeated three times. Figure 3: miR-205 regulates DNA damage repair and radiosensitivity through ZEB1 and Ubc13. ( a ) γH2AX and 4',6-diamidino-2-phenylindole (DAPI) staining of SUM159-P2 cells transfected with miR-205 or scramble control oligonucleotides, 24 h after 6-Gy IR. Scale bar, 20 μm. ( b ) HR repair assays of U2OS_DR-GFP cells transfected with miR-205 alone or in combination with ZEB1. n =3 wells per group. ( c ) Immunoblotting of ZEB1, Ubc13, BRCA1 and GAPDH in SUM159-P0 cells transfected with miR-205 mimics or the miR-205 inhibitor. ( d ) Luciferase activity of the wild-type (UTR-WT) or mutant (UTR-mut.) Ubc13 3′ UTR reporter gene in 293T cells transfected with the miR-205-expressing or empty vector. n =3 wells per group. ( e ) Immunoblotting of K63-linked polyubiquitin chains, Ubc13 and GAPDH in SUM159-P0 and SUM159-P2 cells. ( f ) Clonogenic survival assays of SUM159-P2 cells transfected with Ubc13 siRNA. n =3 wells per group. ( g ) Top: clonogenic survival assays of miR-205-transduced SUM159-P2 cells with or without ectopic expression of ZEB1 and Ubc13. Bottom: immunoblotting of ZEB1, Ubc13 and GAPDH. n =3 wells per group. ( h ) HR repair assays of U2OS_DR-GFP cells transfected with miR-205 alone or in combination with ZEB1 or Ubc13, or both. n =3 wells per group. Data in b , d , f , g , h are the mean of biological replicates from a representative experiment, and error bars indicate s.e.m. Statistical significance was determined by a two-tailed, unpaired Student’s t -test. The experiments were repeated three times. Full size image Among the targets predicted by both the TargetScan [42] and PicTar [43] programmes for miR-205, Ubc13 and BRCA1 play essential roles in HR repair [44] , [45] . In SUM159-P0 cells, transfection of the miR-205 antisense inhibitor increased ZEB1 and Ubc13 protein levels, and transfection of miR-205 mimics downregulated ZEB1 and Ubc13, whereas BRCA1 protein level was not altered by either transfection ( Fig. 3c ). Similar effects were also observed in MDA-MB-231 cells ( Supplementary Fig. 3b ). Moreover, the activity of a luciferase reporter fused to a wild-type Ubc13 3′ untranslated region (UTR), but not that of a reporter fused to a mutant Ubc13 3′ UTR with the mutated miR-205-binding site ( Supplementary Fig. 3c ), was significantly reduced by the overexpression of miR-205 ( Fig. 3d ), which confirmed Ubc13 as a direct target of this miRNA. Similar to the expression pattern of ZEB1 (ref. 41 ), Ubc13 protein was significantly upregulated in SUM159-P2 cells relative to the parental SUM159 cells ( Fig. 3e ). Consistent with the previous finding that Ubc13 promotes HR-mediated DSB repair by conjugating lysine 63 (K63)-linked ubiquitin chains to a number of target proteins including H2AX and PCNA [44] , [46] , [47] , K63-linked polyubiquitination was enriched in SUM159-P2 cells ( Fig. 3e ). We examined whether Ubc13 is a functional target of miR-205 in addition to ZEB1. Two independent Ubc13 siRNAs both increased the radiosensitivity of SUM159-P2 cells ( Fig. 3f ), which recapitulated the effect of miR-205 ( Fig. 1d ). Next, we re-expressed ZEB1 and Ubc13, singly or in combination, in miR-205-overexpressing SUM159-P2 or U2OS cells. Either ZEB1 or Ubc13 alone partially restored radioresistance and HR repair, and co-expression of ZEB1 and Ubc13 led to a nearly complete rescue ( Fig. 3g,h and Supplementary Fig. 3d ). Collectively, these results suggest that miR-205 inhibits HR-mediated DNA damage repair and radioresistance by targeting ZEB1 and Ubc13 . Radiation downregulates miR-205 through ATM and ZEB1 We sought to determine the mechanism by which miR-205 is downregulated in SUM159-P2 cells. Recent studies have revealed a feedback loop whereby the miR-200 family of miRNAs directly targets ZEB1 (ref. 29 ) and ZEB1 represses the transcription of miR-200 genes [48] . We asked whether ZEB1 is also a transcriptional repressor of miR-205. Indeed, the knockdown of ZEB1 in SUM159-P2 cells increased miR-205 expression levels by 63-fold ( Fig. 4a ). Moreover, Zeb1 -deficient mouse embryonic fibroblasts (MEFs) exhibited prominent upregulation of miR-205 ( Fig. 4b ). 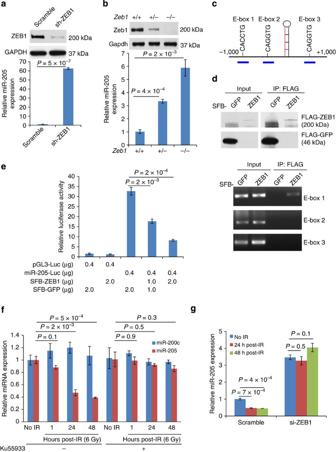Figure 4: Radiation downregulates miR-205 expression through ZEB1 and ATM. (a) Immunoblotting of ZEB1 and GAPDH (top) and quantitative PCR (qPCR) of miR-205 (bottom) in SUM159-P2 cells transduced with ZEB1 shRNA.n=3 samples per group. (b) Immunoblotting of Zeb1 and Gapdh (top) and qPCR of miR-205 (bottom) inZeb1+/+,Zeb1+/−andZeb1−/−MEFs.n=3 samples per group. (c) Humanmir-205genomic locus. The three short blue lines represent PCR amplicons specific for three E-box elements. (d) Top: 293T cells were transfected with SFB-GFP or SFB-ZEB1, immunoprecipitated with the FLAG antibody and immunoblotted with the FLAG antibody. Bottom: ChIP assays of 293T cells transfected with SFB-GFP or SFB-ZEB1. PCR was performed with primers specific for E-box elements 1, 2 and 3. (e) Activity of a luciferase reporter fused to the putative humanmir-205promoter in 293T cells transfected with SFB-GFP or SFB-ZEB1.n=3 wells per group. (f) qPCR of miR-205 and miR-200c in irradiated SUM159-P0 cells with or without pretreatment with the ATM inhibitor Ku55933 (10 μM, 1 h).n=3 samples per group. (g) qPCR of miR-205 in SUM159-P0 cells transfected with ZEB1 siRNA or scramble control oligonucleotides. Cells were treated with 6-Gy IR.n=3 samples per group. Data ina,b,e,f,gare the mean of biological replicates from a representative experiment, and error bars indicate s.e.m. Statistical significance was determined by a two-tailed, unpaired Student’st-test. The experiments were repeated three times. Figure 4: Radiation downregulates miR-205 expression through ZEB1 and ATM. ( a ) Immunoblotting of ZEB1 and GAPDH (top) and quantitative PCR (qPCR) of miR-205 (bottom) in SUM159-P2 cells transduced with ZEB1 shRNA. n =3 samples per group. ( b ) Immunoblotting of Zeb1 and Gapdh (top) and qPCR of miR-205 (bottom) in Zeb1 +/+ , Zeb1 +/− and Zeb1 −/− MEFs. n =3 samples per group. ( c ) Human mir-205 genomic locus. The three short blue lines represent PCR amplicons specific for three E-box elements. ( d ) Top: 293T cells were transfected with SFB-GFP or SFB-ZEB1, immunoprecipitated with the FLAG antibody and immunoblotted with the FLAG antibody. Bottom: ChIP assays of 293T cells transfected with SFB-GFP or SFB-ZEB1. PCR was performed with primers specific for E-box elements 1, 2 and 3. ( e ) Activity of a luciferase reporter fused to the putative human mir-205 promoter in 293T cells transfected with SFB-GFP or SFB-ZEB1. n =3 wells per group. ( f ) qPCR of miR-205 and miR-200c in irradiated SUM159-P0 cells with or without pretreatment with the ATM inhibitor Ku55933 (10 μM, 1 h). n =3 samples per group. ( g ) qPCR of miR-205 in SUM159-P0 cells transfected with ZEB1 siRNA or scramble control oligonucleotides. Cells were treated with 6-Gy IR. n =3 samples per group. Data in a , b , e , f , g are the mean of biological replicates from a representative experiment, and error bars indicate s.e.m. Statistical significance was determined by a two-tailed, unpaired Student’s t -test. The experiments were repeated three times. Full size image ZEB1 is known to bind to E-box elements and act as a transcriptional repressor through recruitment of co-repressors CTBP1 and CTBP2 (refs 49 , 50 ). We examined the genomic sequences flanking the human miR-205 stem-loop (pre-miR-205) and identified three E-boxes, at −417 bp (E-box 1), −186 bp (E-box 2) and +550 bp (E-box 3; Fig. 4c ). We designed PCR amplicons to assay for the presence of these three putative binding sites in chromatin immunoprecipitates. This experiment revealed that either overexpressed ( Fig. 4d ) or endogenous ( Supplementary Fig. 4a ) ZEB1 protein bound to E-box 1 located 417 bp upstream of the start site of pre-miR-205, but not to E-box 2 or E-box 3 ( Fig. 4d ). Moreover, SUM159-P2 exhibited increased occupancy of E-box 1 by endogenous ZEB1 than SUM159-P0 cells ( Supplementary Fig. 4a ). In addition, luciferase reporter assays demonstrated that the overexpression of ZEB1 significantly repressed the activity of the putative mir-205 promoter ( Fig. 4e ). To confirm that endogenous ZEB1 represses miR-205 expression, we compared the reporter activity in SUM159-P0 versus SUM159-P2 cells ( Supplementary Fig. 4b ), in MDA-MB-231 versus MCF-7 cells ( Supplementary Fig. 4c ), and in SUM159-P2 ( Supplementary Fig. 4d ) or MDA-MB-231 ( Supplementary Fig. 4e ) cells with or without knockdown of ZEB1. In all cases, the reporter activity inversely correlated with the expression level of endogenous ZEB1 ( Supplementary Fig. 4b–e ). ATM kinase is a key sensor of DNA damage especially DSBs [51] . We previously found that ATM-mediated phosphorylation of ZEB1 at serine 585 is crucial for IR-induced stabilization of ZEB1 protein [41] . To determine whether IR regulates miR-205 expression through ATM and ZEB1, we irradiated SUM159-P0 cells that had been treated with an ATM kinase inhibitor (Ku55933) or transfected with ZEB1 siRNA. We found that miR-205, but not miR-200c, was significantly downregulated 24 h after irradiation, which was accompanied by upregulation of ZEB1 ( Fig. 4f and Supplementary Fig. 4f ). Notably, either inhibition of ATM ( Fig. 4f ) or depletion of ZEB1 ( Fig. 4g ) completely abolished the downregulation of miR-205 by IR. Taken together with our previous findings [41] , these results support a model in which ATM phosphorylates and stabilizes ZEB1 on irradiation, and ZEB1 in turn represses its own negative regulator, miR-205, leading to further upregulation of ZEB1, increased Ubc13 levels and enhanced DNA repair and radioresistance ( Fig. 5 ). Importantly, our study identified miR-205 mimics as a candidate radiosensitizing agent. 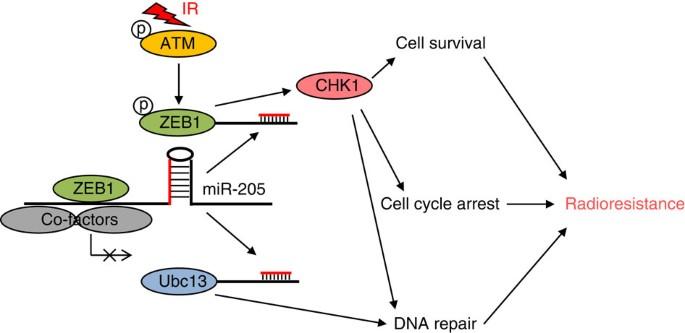Figure 5: The working model of regulation of radiosensitivity and DNA damage repair by miR-205. In response to IR, ATM kinase is rapidly activated, which phosphorylates and stabilizes ZEB1, leading to upregulation of CHK1. In parallel, ZEB1 downregulates its own negative regulator, miR-205, leading to further upregulation of ZEB1, increased Ubc13 expression and enhanced DNA repair and radioresistance. Figure 5: The working model of regulation of radiosensitivity and DNA damage repair by miR-205. In response to IR, ATM kinase is rapidly activated, which phosphorylates and stabilizes ZEB1, leading to upregulation of CHK1. In parallel, ZEB1 downregulates its own negative regulator, miR-205, leading to further upregulation of ZEB1, increased Ubc13 expression and enhanced DNA repair and radioresistance. Full size image Constitutive activation of DNA damage response components has been observed in radioresistant breast tumours [1] . To improve the outcomes in these cases, many groups are dedicated to identifying the agents that target DNA damage response pathways which mediate radioresistance. Although numerous proteins are known to regulate the response to radiation, few of them can be targeted therapeutically. This is where miRNAs could offer new possibilities. The ability of miRNAs to act as negative gene regulators allows them to modulate signalling pathways that regulate multiple cellular processes, including the response to radiation. Consequently, they have the potential to be used as either radiosensitizers or radioprotectors. Using a radioresistant model and an unbiased miRNA expression profiling approach, we identified miR-205 as the top downregulated miRNA in radioresistant breast cancer cells. Interestingly, miR-205 and ZEB1 negatively regulate each other and play opposing roles in regulating DNA damage response and tumour radiosensitivity. In addition to downregulating miR-205, ZEB1 has been shown to repress miR-200c expression [48] , and indeed, we observed upregulation of both miR-205 ( Fig. 4b ) and miR-200c (data not shown) in Zeb1 knockout MEFs. However, only miR-205, but not miR-200c, was downregulated by IR ( Fig. 4f ). One possibility is that ZEB1 may recruit a specific co-repressor to the mir-205 promoter but not to the mir-200c promoter in this context. In fact, it has been shown that ZEB1 recruits distinct transcriptional co-factors in different contexts. For example, Postigo et al. [52] reported that ZEB1 normally recruits the co-repressor CtBP1 but not co-activators p300 and P/CAF; however, in response to transforming growth factor-β, recruitment of p300-P/CAF leads to the displacement of CtBP1 from ZEB1, which in turn promotes the formation of a p300-SMAD transcriptional complex and activates transforming growth factor-β-responsive genes. Moreover, it should be noted that the transcription factor p63 (ref. 53 ) and the polycomb protein Mel-18 (ref. 54 ) have been shown to regulate the transcription of mir-205 . Thus, ZEB1 might not be the only regulator of miR-205 expression in response to radiation. Upregulation of ZEB1 and downregulation of miR-205 have been found in human breast tumours [55] , [56] , [57] , [58] and other clinical cancer types [59] , [60] , [61] , [62] . Taken together with our previous finding [41] , our results raise the caution that radiation treatment may lead to upregulation of ZEB1, downregulation of miR-205 and therapy-induced radioresistance. On the basis of our data, ZEB1-targing agents, like the miR-205 mimics, represent a new class of radiosensitizing agents. Cell culture MEFs were isolated from Zeb1 -deficient embryos, genotyped and cultured in DMEM medium supplemented with 10% fetal bovine serum and 1% penicillin and streptomycin [63] . The 293T, MDA-MB-231, MCF-7, T47D and A549 cell lines were from ATCC and cultured under conditions specified by the manufacturer. The SUM159 cell line was from S. Ethier and cultured as described ( http://www.asterand.com/Asterand/human_tissues/159PT.htm ). The HMLE cell line was from R.A. Weinberg’s lab stock and cultured in complete Mammary Epithelial Cell Growth Medium (MEGM from Lonza). The DR-GFP-expressing U2OS cell line was from J. Chen’s lab stock and cultured in RPMI 1640 medium supplemented with 10% FBS and 1% penicillin and streptomycin. Plasmids and shRNA The ZEB1 expression constructs were from R.A. Weinberg. The following short hairpin RNA (shRNA) and ORF clones were from Open Biosystems through MD Anderson’s shRNA and ORFeome Core: human ZEB1 shRNA, V3LHS-356186 (5′-AGATTTACTGTGCTGTCCT-3′); human Ubc13 (UBE2N) ORF, PLOHS_100006526. The human mir-205 genomic region, which contains the three putative ZEB1-binding sites (E-boxes 1, 2 and 3) and spans from 602 bp upstream of the start site of pre-miR-205 to 710 bp downstream of the start site of pre-miR-205, was PCR amplified from normal genomic DNA and cloned into the pGL3-Basic vector, using the following cloning primers: forward, 5′-CCCTCGAGGTTGTGGTTTTTCCTGAG-3′; reverse, 5′-CCAAGCTTCACTTAAATTTTATTTACATTTAC-3′. A Ubc13 3′ UTR fragment (500 bp) was cloned into the pMIR-REPORT vector, using the following cloning primers: forward, 5′-CTTGACTAGTATTGATACGATCATCAAGTGTGC-3′; reverse, 5′-CTAGAAGCTTGCGTCTAAATAAAGTTAGACTTGGCT-3′. The vectors used in this study are listed in Supplementary Table 2 . siRNA oligonucleotides Two individual siRNAs that target human Ubc13 were purchased from Sigma (si-Ubc13 #1, SASI_Hs02_00326304; si-Ubc13 #2, SASI_Hs02_00326305). The on-target plus siRNA that targets human ZEB1 was purchased from Dharmacon (J-006564-10-0005). Cells were transfected with 150 nM of the indicated oligonucleotide using the Oligofectamine reagent (Invitrogen). Forty-eight hours after siRNA transfection, cells were used for functional assays, and the remaining cells were harvested for western blot analysis. RNA isolation and real-time RT-PCR Total RNA, inclusive of small RNAs, was isolated using the mirVana miRNA Isolation Kit (Ambion). Quantification of the mature form of miRNAs was performed using the TaqMan MicroRNA Assay Kit (Applied Biosystems) according to the manufacturer’s instructions, and the U6 small nuclear RNA was used as an internal control. Real-time PCR and data collection were performed on a CFX96 instrument (Bio-Rad). Human apoptosis miRNA PCR array analysis The Human Apoptosis miScript miRNA PCR Array, which profiles the expression of 84 miRNAs that regulate programmed cell death by inhibiting pro-apoptotic and anti-apoptotic gene expression, was used to compare SUM159-P2 with SUM159-P0 cells according to the manufacturer’s instructions ( http://www.sabiosciences.com/mirna_pcr_product/HTML/MIHS-114Z.html ). In brief, total RNA was extracted and reverse transcribed into cDNA using a miScript II Reverse Transcription Kit (Qiagen). The cDNA was combined with an RT [2] SYBR Green qPCR Master Mix (Qiagen), and then equal aliquots of this mixture (25 μl) were added to each well of the same PCR Array plate that contained the predispensed gene-specific primer sets. Real-time PCR and data collection were performed on a CFX96 instrument (Bio-Rad). Luciferase reporter assay Cells of 50% confluence in 24-well plates were transfected using Fugene 6 (Roche). The firefly luciferase reporter gene construct (400 ng) and the pRL-SV40 Renilla luciferase construct (1 ng, for normalization) were used for cotransfection, with or without 1–2 μg of the SFB-ZEB1 construct. Cell extracts were prepared 24 h after transfection, and the luciferase activity was measured using the Dual-Luciferase Reporter Assay System (Promega). Immunoblotting Western blot analysis was performed with precast gradient gels (Bio-Rad) using standard methods. In brief, cells were lysed in the RIPA buffer containing protease inhibitors (Roche) and phosphatase inhibitors (Sigma). Proteins were separated by SDS–polyacrylamide gel electrophoresis and blotted onto a nitrocellulose membrane (Bio-Rad). Membranes were probed with the specific primary antibodies, followed by peroxidase-conjugated secondary antibodies. The bands were visualized by chemiluminescence (Denville Scientific). The following antibodies were used: antibodies to ZEB1 (1:1000, Bethyl Laboratories, A301-922A), γH2AX (1:1000, Cell Signaling Technology, 2577), K63-linkage specific polyubiquitin (1:1000, Cell signaling Technology, 12930), BRCA1 (1:1000, Bethyl Laboratories, A300-000A), Ubc13 (1:1000, Cell Signaling Technology, 4919), FLAG (1:5000, Sigma, F3165) and GAPDH (1:3000, Thermo, MA5-15738). The ImageJ program ( http://rsbweb.nih.gov/ij/download.html ) was used for densitometric analysis of western blots, and the quantification results were normalized to the loading control. Uncropped images of blots are shown in Supplementary Fig. 5 . Immunofluorescence Cells were cultured in chamber slides overnight and fixed with 3.7% formaldehyde in PBS for 20 min at 4 °C, followed by permeabilization with 0.5% Triton-X-100 in PBS for 30 min. Cells were then blocked for non-specific binding with 10% goat serum in PBS and Tween-20 (PBST) overnight, and incubated with the anti-γH2AX antibody (1:300, 1:1,000, Millipore, 07-164) for 1 h at 37 °C, followed by incubation with Alexa Fluor 594 goat anti-mouse IgG (1:400, Invitrogen, A11005) for 1 h at 37 °C. Cover slips were mounted on slides using anti-fade mounting medium with 4′,6-diamidino-2-phenylindole. Immunofluorescence images were acquired on a Zeiss Axio Observer Z1 fluorescence microscope. Chromatin immunoprecipitation (ChIP) assay ChIP was performed with SUM159-P0, SUM159-P2, or 293T cells transfected with SFB-GFP control or SFB-ZEB1, by using a ChIP Assay Kit (Millipore, 17–295) according to the manufacturer’s instructions. After immunoprecipitation with the ZEB1 antibody (1:100, Bethyl Laboratories, A301-922A) or FLAG antibody-conjugated beads (Sigma, M8823), protein–DNA crosslinks were reversed and DNA was purified to remove the chromatin proteins and used for PCR. The PCR primers are: E-box 1, 5′-GGCCTTGGTAAGCAAGCTCAG-3′ (forward) and 5′-CTCGGTGTGGTTGGTCCTTTC-3′(reverse); E-box 2, 5′-TGGCCCCACAGACCCACCT-3′ (forward) and 5′-CATCCTCCAAGGAGGCTGCA-3′ (reverse); E-box 3, 5′-AACTGAGACATGAACTTG-3′ (forward) and 5′-AGGGTTCCTTGCTGATTG-3′ (reverse). Clonogenic assay Equal numbers of cells were plated in 10-cm tissue culture dishes at a clonogenic density (500 cells per dish) and irradiated by using a JL Shepherd Mark I-68A 137Cs irradiator with the indicated doses. Cells were incubated for 10–14 days. Colonies were stained with crystal violet and counted using a Gel Doc EZ Imager instrument (Bio-Rad) with the Quantity One software. The survival fraction was calculated as: (number of colonies/number of cells plated) irradiated /(number of colonies/number of cells plated) non-irradiated . HR repair assay A U2OS cell clone stably expressing an HR repair reporter was described previously [40] . In brief, 2 days after transfection with the indicated miRNA mimics, 1 × 10 6 U2OS cells expressing the HR repair reporter were electroporated with 10 μg of pCBASce, an I-SceI expression vector described previously [64] . Cells were harvested 2 days after electroporation and subjected to flow cytometry analysis to determine the percentage of GFP-positive cells resulting from HR-based repair of I-SceI-induced DSBs. Tumour radiosensitivity study Animal experiments were performed as previously described [65] in accordance with a protocol approved by the Institutional Animal Care and Use Committee of MD Anderson Cancer Center, and mice were killed when they met the institutional euthanasia criteria for tumour size and overall health condition. When used in a power calculation, our sample size predetermination experiments indicated that five mice per group can identify the expected effect of miR-205 on tumour radiosensitivity ( P <0.05) with 100% power. Solitary tumour xenografts were produced in the muscle of the right hind limb of 3-month-old female athymic nude mice (NCR Nu/Nu) by inoculation of 3 × 10 6 SUM159-P2 cells. Mice were randomly assigned to no treatment or treatment groups. Radiation treatment was initiated when tumours grew to 8.0 mm (range: 7.7–8.2 mm) in diameter. Single doses (15 Gy once) were delivered to the tumour-bearing limb of mice using a small-animal irradiator (Co-V, Theratron 780; MDS Nordion, Ottawa, Ontario) with a cobalt Co 60 source (field size, 10 × 10 cm; source axis distance, 64.9 cm), at a dose rate of 0.955 Gy min −1 . During irradiation, unanesthetized mice were mechanically immobilized in a jig so that the tumour was exposed in radiation field but the animal’s body was shielded from radiation exposure. Three mutually orthogonal diameters of the tumour were measured every other day with a caliper, and the mean value was calculated and used as the tumour diameter. An investigator (L.W.) who measured the tumour size was blinded to the group allocation during all animal experiments and outcome assessment. General linear model multivariate analysis was performed to determine statistical significance using the SPSS 14.0 software package. Liposomal miRNA preparation and in vivo treatment Nanoliposomal miRNA mimics were prepared and used as previously described [36] . In brief, miRNA oligonucleotides and DOPC were mixed in the presence of excess tertiary butanol at a ratio of 1:10 (miRNA:DOPC). Before in vivo administration, the preparation was hydrated with normal 0.9% saline (200 μl per mouse) for subcutaneous injection. One week before tumours grew to 8.0 mm (range: 7.7–8.2 mm) in diameter, mice were injected with 250 μg kg −1 of DOPC-encapsulated miR-205 mimics or a scramble control. Injection was performed twice per week till the end point. Statistical analysis Each experiment was repeated three times or more. Unless otherwise noted, data are presented as mean±s.e.m, and Student’s t -test (unpaired, two-tailed) was used to compare two groups for independent samples. The data analysed by t -test meet normal distribution; we used an F-test to compare variances, and the variances are not significantly different. Therefore, when using an unpaired t -test, we assumed equal variance, and no samples were excluded from the analysis. P <0.05 was considered statistically significant. How to cite this article: Zhang, P. et al. miR-205 acts as a tumor radiosensitizer by targeting ZEB1 and Ubc13. Nat. Commun. 5:5671 doi: 10.1038/ncomms6671 (2014). Accession codes: The miRNA qPCR array data have been deposited in the Gene Expression Omnibus database under accession code GSE62511 .